Magnon transistor for all-magnon data processing An attractive direction in next-generation information processing is the development of systems employing particles or quasiparticles other than electrons—ideally with low dissipation—as information carriers. One such candidate is the magnon: the quasiparticle associated with the eigen-excitations of magnetic materials known as spin waves. The realization of single-chip all-magnon information systems demands the development of circuits in which magnon currents can be manipulated by magnons themselves. Using a magnonic crystal—an artificial magnetic material—to enhance nonlinear magnon–magnon interactions, we have succeeded in the realization of magnon-by-magnon control, and the development of a magnon transistor. We present a proof of concept three-terminal device fabricated from an electrically insulating magnetic material. We demonstrate that the density of magnons flowing from the transistor’s source to its drain can be decreased three orders of magnitude by the injection of magnons into the transistor’s gate. A field-effect transistor, which is the key element of modern complementary metal oxide semiconductor (CMOS) technology, is used in microprocessors, static random access memory and other digital logic circuits. Nevertheless, the future of CMOS is not clear, since both the miniaturization of single-element sizes and the operational speed will reach their ultimate limits in the near future [1] . Therefore, one of the primary tasks facing modern science is the search for alternative concepts to CMOS. Distinct achievements in this direction are the development of transistors based on carbon nanotubes and graphene nanoribbons [2] , [3] , spin torque transistors [4] , [5] as well as three-dimensional spintronic circuits [6] . However, these approaches do not resolve another drawback of CMOS technology: the generation of waste heat during switching that is responsible for an increase in the power consumption of CMOS devices. Moreover, the waste heat increases with increasing data-processing speed due to the high switching frequencies. This fundamental drawback is inherent not only in CMOS, but in electronics in general since it is associated with a translational motion of electrons. Thus, there is a strong need for the development of new particle-less technologies for data transport and processing. Magnons, which are the quanta of spin waves [7] , [8] , are excellent candidates for carriers in such technologies. Magnonics, the field of science dealing with magnon-based data operations [9] , [10] , [11] , [12] , encompasses a full spectrum of phenomena used in general wave-based signal processing [13] , [14] , [15] , [16] , [17] . The data can be coded into magnon phase or density and processed using wave effects such as interference. This approach has already been realized in spin-wave logic gates performing XNOR and NAND operations [18] , [19] , [20] , [21] . The main drawback of these gates is that the input data were coded in a form of direct current electric pulses manipulating magnon phases, while the output signal was carried by the magnons themselves. Obviously, that made it impossible to combine two logic gates without additional magnon-to-voltage converters. Moreover, the processing of large amounts of data has to be made on the same magnetic chip exclusively within the magnonic system. This fact stimulated a search for a way to control one magnon by another magnon and for the development of the all-magnon device presented in this paper. In addition, recent discoveries in the fields of spin transfer torque [22] , [23] , spin pumping and inverse spin Hall effects [24] , [25] , [26] made it possible to perform interconversion of currents of magnons to electron-carried spin- and charge-currents and combine, in such a way, magnonic circuits with spintronic or CMOS devices. Here we report on the realization of an insulator-based magnon transistor. The information is carried and processed in this three-terminal device using magnons and is fully decoupled from free electrons. The device demonstrated here has the potential to be scaled down [27] to the sub-ten nanometer scale using exchange magnons [26] , [28] . Regarding frequency, there is large potential for ultra-fast data processing since magnon frequencies can reach up into the THz range [28] , [29] , [30] . Transistor’s design The magnon transistor is shown schematically in Fig. 1a . Its main element is an artificial magnetic material—a magnonic crystal [31] , [32] , [33] , [34] , [35] , [36] , [37] , [38] designed in the form of a yttrium iron garnet (YIG) strip with periodic modulation of its thickness [33] , [38] : in our demonstrator, an array of 20 parallel grooves was etched into the surface of the strip (see Methods). The flow of magnons propagating through the crystal is partially (around one per cent [33] ) reflected from each groove and the influence of the grooves is negligible for most of the magnons. Nevertheless, the magnons which have wavelengths satisfying the Bragg conditions k a = m·π / a (where m is an integer and a =300 μm is the crystal lattice constant) will be resonantly scattered back resulting in the generation of rejection bands (band gaps) in a spin-wave spectrum over which magnon propagation is fully prohibited [10] , [11] , [12] , [31] , [32] , [33] , [34] , [35] , [36] , [37] , [38] . The measured magnonic-crystal transmission spectrum shows pronounced band gaps and is displayed in the inset of Fig. 2b . 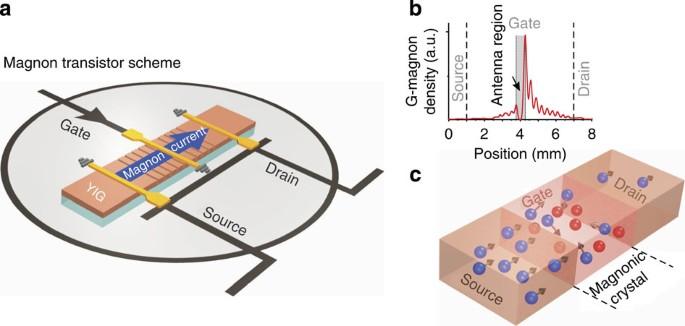Figure 1: Schematic of the magnon transistor, spatial distribution of the gate magnons and the transistor’s operational principle. (a) The transistor is based on a magnonic crystal designed in the form of a yttrium iron garnet (YIG) film with an array of parallel grooves at its surface. The magnons are injected into the transistor’s source and are detected at its drain using microstrip antennas (other methods of injection, for example, via magnon conduits40, might also work). The magnons that control the source-to-drain magnon current are injected directly into the magnonic crystal (transistor’s gate) using an identical antenna. (b) Brillouin light scattering spectroscopy has been used to measure the spatial distribution of the gate magnons in the absence of source magnons. Strong magnon localization and the formation of a standing-wave-like intensity profile is visible. The asymmetry of the intensity profile might be related to the injection mechanism by means of the microstrip antenna influenced by the dynamic demagnetizing field of the adjacent grooves. (c) A magnon transistor allows for the suppression of the source-to-drain magnon current (shown with blue spheres) via the injection of the gate magnons (red spheres) into the gate region. A nonlinear four-magnon scattering mechanism is responsible for the transistor’s operational principle: when magnons from the transistor’s source enter the gate region, they are scattered by the gate magnons and, thus, reach the transistor’s drain with attenuation. The high degree of gate magnon localization inside the crystal consequently leads to high scattering probabilities provided by the magnonic crystal, which, hence, serves as an enhancer of the nonlinear effects. The secondary magnons generated due to the scattering have large wavevectors and small group velocities that prohibit their flow out of the gate region. Figure 1: Schematic of the magnon transistor, spatial distribution of the gate magnons and the transistor’s operational principle. ( a ) The transistor is based on a magnonic crystal designed in the form of a yttrium iron garnet (YIG) film with an array of parallel grooves at its surface. The magnons are injected into the transistor’s source and are detected at its drain using microstrip antennas (other methods of injection, for example, via magnon conduits [40] , might also work). The magnons that control the source-to-drain magnon current are injected directly into the magnonic crystal (transistor’s gate) using an identical antenna. ( b ) Brillouin light scattering spectroscopy has been used to measure the spatial distribution of the gate magnons in the absence of source magnons. Strong magnon localization and the formation of a standing-wave-like intensity profile is visible. The asymmetry of the intensity profile might be related to the injection mechanism by means of the microstrip antenna influenced by the dynamic demagnetizing field of the adjacent grooves. ( c ) A magnon transistor allows for the suppression of the source-to-drain magnon current (shown with blue spheres) via the injection of the gate magnons (red spheres) into the gate region. A nonlinear four-magnon scattering mechanism is responsible for the transistor’s operational principle: when magnons from the transistor’s source enter the gate region, they are scattered by the gate magnons and, thus, reach the transistor’s drain with attenuation. The high degree of gate magnon localization inside the crystal consequently leads to high scattering probabilities provided by the magnonic crystal, which, hence, serves as an enhancer of the nonlinear effects. The secondary magnons generated due to the scattering have large wavevectors and small group velocities that prohibit their flow out of the gate region. 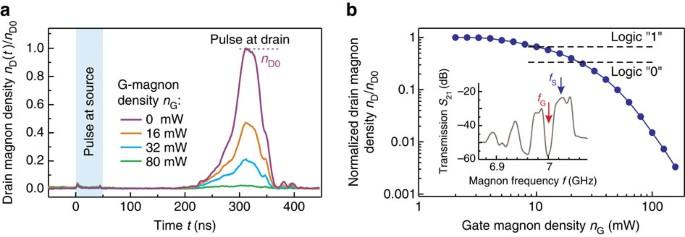Figure 2: Suppression of the source-to-drain magnon current by gate magnons. The inset inbshows the magnon transmission characteristic through the magnonic crystal as a function of the magnon frequency. The frequency of the magnons injected into the transistor’s sourcefS=7.025 GHz is chosen to be in the transmission region required for supporting their distortion-free propagation through the crystal. Consequently, the frequency of the magnons injected into the gatefG=7 GHz is chosen to be in the centre of the first band gap ensuring the localization of these magnons inside the crystal. (a) The time evolution of the signal at the transistor’s drain carried by 50-ns long magnon packets injected into the transistor’s source at the timet=0 ns. A magnon packet requires about 300 ns to travel the 8-mm distance to the drain. The injection of magnons into the gate region (nG>0) results in the suppression of the travelling magnon packet density while preserving the packet shape. (b) To show the degree of the suppression, the drain magnon densitynDnormalized to the original valuenD0is presented as a function of the gate magnon densitynGon a logarithmic scale. A suppression of about three orders of magnitude is achieved. The horizontal-dashed lines split the densitynDat the transistor’s drain to the signals corresponding to a logic ‘1’ (the relative amplitude of the signalnD/nD0is larger than 2/3) and to a logic ‘0’ (nD/nD0<1/3). Full size image Figure 2: Suppression of the source-to-drain magnon current by gate magnons. The inset in b shows the magnon transmission characteristic through the magnonic crystal as a function of the magnon frequency. The frequency of the magnons injected into the transistor’s source f S =7.025 GHz is chosen to be in the transmission region required for supporting their distortion-free propagation through the crystal. Consequently, the frequency of the magnons injected into the gate f G =7 GHz is chosen to be in the centre of the first band gap ensuring the localization of these magnons inside the crystal. ( a ) The time evolution of the signal at the transistor’s drain carried by 50-ns long magnon packets injected into the transistor’s source at the time t =0 ns. A magnon packet requires about 300 ns to travel the 8-mm distance to the drain. The injection of magnons into the gate region ( n G >0) results in the suppression of the travelling magnon packet density while preserving the packet shape. ( b ) To show the degree of the suppression, the drain magnon density n D normalized to the original value n D0 is presented as a function of the gate magnon density n G on a logarithmic scale. A suppression of about three orders of magnitude is achieved. The horizontal-dashed lines split the density n D at the transistor’s drain to the signals corresponding to a logic ‘1’ (the relative amplitude of the signal n D / n D0 is larger than 2/3) and to a logic ‘0’ ( n D / n D0 <1/3). Full size image The YIG magnonic crystal is magnetized along its long axis, and thus along the magnon propagation direction, by an applied biasing magnetic field B =177 mT. This provides the conditions for the excitation and propagation of backward volume magnetostatic waves [8] , which are known for their high scattering efficiency in grooved magnonic crystal [39] . In order to inject the magnons into and to collect them from the transistor, as well as to control them by the gate magnons, three identical microstrip antennas [10] are placed at equal distances 4 mm apart. The antenna that injects magnons into the transistor’s gate is placed at the middle of the magnonic crystal area, while the source and the drain antennas are placed outside in the non-structured YIG film areas. It has to be emphasized that all antennas are only used as an instrument for magnon injection and detection, and thus they are not part of the transistor. In forthcoming all-magnon circuits, the antennas will be absent and the magnons will be injected into or collected from another magnon data-processing unit via magnon conduits. A promising way for this might be, for example, the usage of T-shaped structures, which allow for the design of two-dimensional magnon circuits [40] . Operational principle of the magnon transistor The operational principle of the transistor is shown in Fig. 1c . The idea is as follows: magnons are injected into the transistor’s source (S-magnons shown in blue in the scheme in Fig. 1c ) at a frequency corresponding to the magnon transmission band, that is, f S =7.025 GHz, see the inset in Fig. 2b . In the case of absence of magnons in the transistor’s gate, the S-magnons propagate towards the drain practically without distortion [33] . Therefore, the density of the magnons at the drain (D-magnons) n D is given by the density of the S-magnons n S with additional consideration being given to magnetic losses due to weak magnon–phonon scattering [8] . In order to manipulate the magnon current flowing from the transistor’s source to the drain, magnons are injected into the gate region (G-magnons, shown in red in Fig. 1c ). The frequency of the G-magnons f G =7 GHz is chosen to be in the centre of the magnonic crystal band gap that prohibits the flow of the G-magnons out of the magnonic crystal area. This confinement allows for a large increase of the G-magnon concentration and, consequently, for an increase in the related efficiency of nonlinear phenomena. The spatial distribution of the G-magnons in the gate region in the absence of S-magnons was measured using the technique of Brillouin Light Scattering [10] , [41] and is shown in Fig. 1b . The localization of the G-magnons in the central part of the gate is clearly visible. Further, the S-magnons injected into the source region, while propagating through the transistor’s gate populated with G-magnons, are scattered and, therefore, are able to reach the transistor’s drain only partially (see Fig. 1c ). To demonstrate this principle experimentally, we applied a pulsed microwave signal of 50-ns duration at time t =0 to the source antenna. The injected S-magnon packets propagate a distance of 8 mm to the transistor’s drain in approximately 300 ns, inducing the output microwave signal at the drain antenna (this value corresponds well with the calculated magnon velocity of 28 km s −1 , which results in a propagation time of 286 ns). The applied rectangular input pulse as well as the transmitted magnon signal, which is slightly distorted from the rectangular shape due to a dispersion spreading, are shown in Fig. 2a . The detected D-magnon density is maximal in the absence of gate magnons, that is, n G =0 mW, and its maximum density is denoted as n D0 . (Please note that for simplicity, we measure the magnon densities in Watts corresponding directly to the power of the microwave signals applied to or measured at the antennas.) The application of a continuous-wave signal to the gate antenna and the injection of the G-magnons result in the suppression of the transmitted signal as shown in the figure. The profile of the transmitted signal subject to suppression remains undisturbed thus ensuring information preservation. For relatively large magnon densities of n G ≥80 mW, almost no magnons are able to propagate through the gate region, and the peak density of the D-magnons (marked as n D ) approaches zero. The dependence of the D-magnon density n D normalized to the original density n D0 is shown in Fig. 2b as a function of the G-magnon density. It can be seen that the suppression increases monotonically with an increase in the G-magnon density and spans almost three orders of magnitude. For the purpose of digital data processing, we use the approach used in CMOS assuming that logic ‘0’ corresponds to the amplitude of the signal smaller than 1/3 of the signal maximum ( n D / n D0 <1/3) and logic ‘1’ corresponds to signals larger than 2/3 ( n D / n D0 >2/3). This approach allows for the minimization of possible errors in definition of the bit state. Figure 2b shows that it is sufficient to inject G-magnons having a density of only 25 mW in order to switch the binary signal from ‘1’ to ‘0’. Underlying physical mechanism In order to determine the physical mechanism responsible for the magnon scattering in the transistor’s gate, we analyse the magnon dispersion characteristics as shown in Fig. 3a . Dispersions are plotted for 40 spin-wave thickness modes propagating along the source-to-drain axis in both directions thus having positive and negative wavenumbers k . The originally injected S-magnons are shown by a blue-filled circle located on the lowest thickness mode having the maximum excitation efficiency. The G-magnons, injected with a Bragg wavenumber of k G =± k a (red-filled circles) propagate in both directions simultaneously until they undergo Bragg scattering. The standing nature of the G-magnons is shown in the figure with a red-dashed horizontal line. 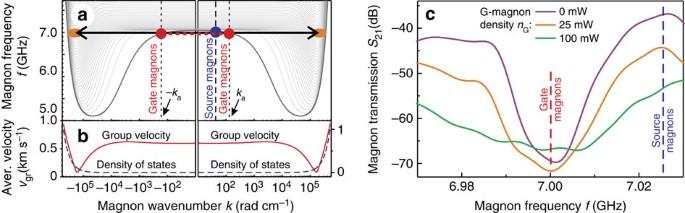Figure 3: The nonlinear phenomena taking place in the transistor’s gate. (a) Magnon dispersion in the 5.5-μm thick YIG film magnetized in-plane with a bias magnetic field of 177 mT. The dispersion of the first 40 thickness modes propagating along and opposite to the magnetic field are shown. The spectral positions of the source and the gate magnons are shown with blue- and red-filled circles, respectively. The standing nature of the gate magnons is shown schematically with a red-dashed horizontal line. The four-magnon scattering processes occur in the high-wavevector regions, which are depicted with orange ellipses. (b) Average group velocity of all modes shown inaobtained as a derivative of their dispersion curves is shown by a solid red line (left scale). The magnons that possess the minimum group velocity have the highest probability to participate in the four-magnon scattering process. The dashed blue line (right scale) shows the normalized density of states, which is proportional to the scattering probability. It is visible that the magnons with wavenumber ≥105rad cm−1(orange ellipses ina) have the highest probability to participate in the four-magnon scattering process. (c) Frequency transmission characteristics of the source-to-drain magnon currents with and without gate magnons are shown. No shift in the band gap and, hence, no effect of a nonlinear decrease of the magnetization37is observed. The suppression of the source-to-drain magnon current in the pass-bands of the magnonic crystal is minimally dependent of the magnon frequency. The specific frequencies of the source and gate magnons are marked with dashed vertical lines. Figure 3: The nonlinear phenomena taking place in the transistor’s gate. ( a ) Magnon dispersion in the 5.5-μm thick YIG film magnetized in-plane with a bias magnetic field of 177 mT. The dispersion of the first 40 thickness modes propagating along and opposite to the magnetic field are shown. The spectral positions of the source and the gate magnons are shown with blue- and red-filled circles, respectively. The standing nature of the gate magnons is shown schematically with a red-dashed horizontal line. The four-magnon scattering processes occur in the high-wavevector regions, which are depicted with orange ellipses. ( b ) Average group velocity of all modes shown in a obtained as a derivative of their dispersion curves is shown by a solid red line (left scale). The magnons that possess the minimum group velocity have the highest probability to participate in the four-magnon scattering process. The dashed blue line (right scale) shows the normalized density of states, which is proportional to the scattering probability. It is visible that the magnons with wavenumber ≥10 5 rad cm −1 (orange ellipses in a ) have the highest probability to participate in the four-magnon scattering process. ( c ) Frequency transmission characteristics of the source-to-drain magnon currents with and without gate magnons are shown. No shift in the band gap and, hence, no effect of a nonlinear decrease of the magnetization [37] is observed. The suppression of the source-to-drain magnon current in the pass-bands of the magnonic crystal is minimally dependent of the magnon frequency. The specific frequencies of the source and gate magnons are marked with dashed vertical lines. Full size image The key issue of nonlinear interactions in magnetic media is the density of magnons [42] . In our case, we have artificially increased the density drastically due to the fact that the G-magnons are not able to leave the magnonic crystal and are all localized under the injecting antenna just in the middle of the gate region (see Fig. 1b ). If the concentration of the G-magnons is high enough, the four-magnon scattering mechanism becomes pronounced [8] , [42] , [43] : an S-magnon collides with a G-magnon creating a pair of secondary magnons, see orange ovals in Fig. 3a . The frequencies f 3 , f 4 and the corresponding wavenumbers k 3 , k 4 of the secondary magnons are determined by the energy and momentum conservation laws: f S + f G = f 3 + f 4 ; k S + k G = k 3 + k 4 . Considering that f S ≈ f G , one might assume that one of the most probable scattering mechanisms is scattering with frequency conservation, that is, f 3 = f 4 =( f S + f G )/2 as is shown in the figure. Nevertheless, we cannot exclude other mechanisms with one of the secondary magnons having a lower and the other one a higher frequency. Taking into account the Bose–Einstein distribution of energies for exchange magnons, it can be shown [8] that the density of states (and thus the four-magnon scattering probability) is proportional to k 3 2 = k 4 2 . This density of states is shown in Fig. 3b demonstrating that the scattering probability increases quadratically with the wavenumber. Further, the group velocity, which is responsible for the flow of energy out of the over-populated magnon zone [44] , also influences the efficiency of the scattering since it determines the concentration of the secondary magnons in the gate region. The average of the group velocity of all modes (presented in Fig. 3a ) is shown in Fig. 3b . Well-pronounced velocity minima are visible for wavenumbers of about ±10 5 rad cm −1 . Thus, magnons with wavenumbers equal to or larger than 10 5 rad cm −1 have the highest probability of participation in four-magnon scattering as shown in Fig. 3a (orange ellipses). Since the magnons having such high wavenumbers are not detectable in our experimental conditions, this conclusion is supported by the experimental fact that we were unable to see any additional magnons at the drain antenna (see Fig. 2a ). We also performed an additional experiment measuring the magnons reflected back from the transistor’s gate region. However, no magnons reflected by G-magnons have been detected at the source antenna corroborating our model. In addition, due to the high efficiency of the observed suppression of the source-to-drain magnon current, we might assume that avalanche-like processes also take place when the secondary magnons generated after scattering play the role of new scatterers for the source magnons. In order to determine the time required for the four-magnon scattering process to develop, we have performed additional experiments with a continuous microwave signal applied to the source antenna and a pulsed control signal at the gate antenna. The results show that the time required for the transistor to be closed decreases rapidly with an increase in the G-magnon density and varies between 170 ns and 70 ns for densities of n G =10 mW and n G =100 mW, respectively. Conversely, the time the system needs to recover increases with increase of n G . However, this dependence is not so pronounced: The fastest opening of the transistor took about 50 ns for n G =10 mW and the slowest 110 ns for n G =100 mW. The four-magnon scattering process is not the only mechanism that might take place in the magnon transistor. With further increase of the magnon density, the YIG saturation magnetization decreases resulting in a shift of the dispersion relation and the magnon spectrum towards lower frequencies [37] . To prove the absence of this mechanism in our experiments, we have measured the magnon transmission spectrum in the presence of G-magnons, see Fig. 3c , where the first band gap and the two neighbouring transmission bands are shown. One can see that a suppression of the magnon transmission, rather than a shift of the band gap as shown in ref. 37 , takes place. This proves that the four-magnon scattering mechanism occurring in the transistor is more efficient and requires smaller magnon densities. Additionally, Fig. 3c shows that no heating effects influence our experiments since these would result in a shift of the band gap [45] . From an applications point of view, the equivalent suppression of the source-to-drain magnon current in the transmission bands independently from the magnon frequency allows for the transistor to operate simultaneously with several source signals separated in frequency. Amplification of magnon-carried signals Semiconductor transistors are widely used not only for logical operations but also for the amplification of electronic signals. Such amplification is based on the control of a large signal applied to the transistor’s source by a weak one at the gate. To demonstrate the possibility of this kind of amplification using our device, we have performed a set of n D ( n G ) measurements for different densities of S-magnons at the signal source. The results are shown in Fig. 4a , where the suppression rate of the source-to-drain magnon current ζ =1− n D / n D0 (where n D and n D0 are the densities of the drain magnons with and without signal at the gate, respectively) is presented as a function of the gate magnon density n G normalized to the source magnon density n S . One sees that the suppression mechanism does not depend on the density of the S-magnons: the same percentage of S-magnons is scattered in the transistor’s gate for a given G-magnon density. This can be considered a good operational characteristic of the device. The vertical-dashed line in Fig. 4a separates two regions with n S being smaller and larger with respect to the gate magnon density n G . It can indeed be observed that a high density of S-magnons can be manipulated by a small density of G-magnons, that is, n G < n S . The lowest n G / n S ratio at which the transistor’s source-to-drain magnon current is influenced by G-magnons is near 0.01 in our experiments. 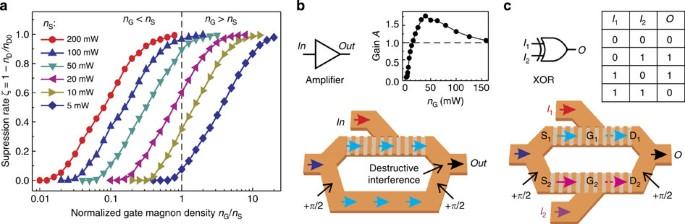Figure 4: Amplification of magnon-carried signals and logic operations. (a) The source-to-drain magnon current suppression rate as a function of the gate magnon densitynGis shown for different source magnon densitiesnS. The densitynGis normalized tonSin order to emphasize the measurements at which the source magnon density is higher than the gate magnon densitynG<nS(left section—see vertical-dashed line). The lowest value ofnG/nSat which the source-to-drain magnon current is influenced by the gate magnons approaches 0.01. (b) A magnonic amplifier based on a Mach–Zehnder interferometer with the magnon transistor embedded in one of its two arms. Aπphase shift inserted by the longer bottom arm ensures the destructive interference of spin waves at the output of the interferometer. The injection of the G-magnons reduces the signal in the upper arm and consequently suppresses the destructive interference. As a result, the temporal evolution of the magnon densitynOat the output reproduces the temporal evolution of the input (gate) densitynI=nG. If the conditionnG<nSis satisfied, the amplificationA=nO/nI>1 is possible. The gainAestimated for our transistor (fornS=200 mW) is shown in the inset ofbas a function ofnG. The maximum gain reaches the value ofAmax=1.8. (c) The operational principle of a XOR logic gate based on the magnon transistor. The feeding magnon currents, which are sent (after splitting) to the transistors’ sources, are independently controlled by the input magnon signalsI1=nG1andI2=nG2applied to the gates. In the case when both input signals are zeroI1=I2=‘0’, the output signalO=‘0’ due to the destructive interference (see the twoπ/2 phase shifts). The application of a signal to only one of the transistors switches off one of the magnon currents (and the destructive interference) resulting inO=‘1’. Finally, switching off both currents results in the absence of magnons at the device’s outputO=‘0’—see the truth table. Figure 4: Amplification of magnon-carried signals and logic operations. ( a ) The source-to-drain magnon current suppression rate as a function of the gate magnon density n G is shown for different source magnon densities n S . The density n G is normalized to n S in order to emphasize the measurements at which the source magnon density is higher than the gate magnon density n G < n S (left section—see vertical-dashed line). The lowest value of n G / n S at which the source-to-drain magnon current is influenced by the gate magnons approaches 0.01. ( b ) A magnonic amplifier based on a Mach–Zehnder interferometer with the magnon transistor embedded in one of its two arms. A π phase shift inserted by the longer bottom arm ensures the destructive interference of spin waves at the output of the interferometer. The injection of the G-magnons reduces the signal in the upper arm and consequently suppresses the destructive interference. As a result, the temporal evolution of the magnon density n O at the output reproduces the temporal evolution of the input (gate) density n I = n G . If the condition n G < n S is satisfied, the amplification A = n O / n I >1 is possible. The gain A estimated for our transistor (for n S =200 mW) is shown in the inset of b as a function of n G . The maximum gain reaches the value of A max =1.8. ( c ) The operational principle of a XOR logic gate based on the magnon transistor. The feeding magnon currents, which are sent (after splitting) to the transistors’ sources, are independently controlled by the input magnon signals I 1 = n G1 and I 2 = n G2 applied to the gates. In the case when both input signals are zero I 1 = I 2 =‘0’, the output signal O =‘0’ due to the destructive interference (see the two π /2 phase shifts). The application of a signal to only one of the transistors switches off one of the magnon currents (and the destructive interference) resulting in O =‘1’. Finally, switching off both currents results in the absence of magnons at the device’s output O =‘0’—see the truth table. Full size image A semiconductor transistor can be embedded into an electronic circuit in such a way that the output signal at the drain is an amplified copy of the input signal at the gate. It is also possible for similar results to be obtained in the case of magnon transistor by using, for example, the magnonic circuit shown schematically in Fig. 4b . It is based on a Mach–Zehnder interferometer with the magnon transistor embedded in one of its two arms. One arm of the interferometer is chosen to be slightly longer in order to induce a π phase shift of the spin wave (see the two π /2 phase shifts in Fig. 4b ) relative to the other arm. As a result, in the case of an input signal equal to zero n I = n G =0 (no G-magnon are injected into the gate), the transistor is open and the destructive interference between the spin waves from both arms leads to an output signal of zero, n O =0. The injection of the G-magnons results in the reduction of the magnonic signal in one of the arms, in the consequent suppression of the destructive interference, and, finally, in the increase of the output signal n O . Thus, the temporal evolution of the density of the magnons at the output of the interferometer n O will reproduce the temporal evolution of the input (gate) density n I (with a short time delay determined by the propagation time of the magnon from the gate to the drain). Important is, that the magnitude of the output magnon signal n O , in this case, is determined by the density of the source magnons n S rather than by the gate magnon density n G . Thus, if the condition n S > n G is fulfilled (see Fig. 4a ), amplification of the magnonic current can be realized. In the approximation of negligible magnetic loss, the output signal n O can be calculated as , where the D-magnon density can be found as n D = n S (1− ζ ). The gain factor A is then given by the ratio A = n O / n I . We have estimated the possible gains of our concrete realization of the transistor for the S-magnon density n S of 200 mW. The gain A is shown in the inset of Fig. 4b as a function of the G-magnon density n G . The gain initially increases with an increase in n G but after reaching some maximum value, it slowly decreases (since if the transistor is practically closed, further increase in n G in all practical terms does not affect the output n O ). The maximum gain factor A achievable in our case is A max =1.8 but it can be considerably improved by an increase in concentrations of G-magnons during the course of further miniaturization/optimization of the transistor. Logic operation on the basis of a magnon transistor The main motivation behind the development of the magnon transistor is the possibility to perform all-magnon processing of digital data. As was shown in the original papers on spin-wave logic gates [18] , [19] , [20] , the usage of Mach–Zehnder interferometer allows for the realization of different types of logic gates. Here we also propose the use of a similar concept, but with two magnon transistors embedded into the arms of the interferometer. The operational principle of such a logic gate is given with the example of a XOR gate and is shown in Fig. 4c . First, the feeding magnon current, which is sent to the interferometer (the left arrow in the figure), is divided into two identical currents. These currents n S1 and n S2 are directly applied to the transistors’ sources S 1 and S 2 and are independently controlled by the input magnon signals I 1 = n G1 and I 2 = n G2 injected into the gates G 1 and G 2 . The input signal I =‘1’ corresponds to the critical gate magnon density n G crit large enough to decrease the magnon density at the drain to the value n D < n D0 /3; the input I =‘0’ means the absence of the gate magnons (the transistor is open). In the case when both input signals are zero I 1 = I 2 =‘0’, the output signal O after the combiner has zero value ‘0’ due to the destructive interference (see permanent π /2 phase shift which appears twice in Fig. 4c ). The application of a signal to only one of the transistors switches off one of the magnon currents and therefore switches off the destructive interference resulting in O =‘1’. Finally, switching off both currents results in the absence of magnons at the devices output O= ‘0’—see the truth table in the Fig. 4c . The great advantage of this kind of wave-based logic gate is that the simple change of the induced phase shifts due to the increased length of the waveguide in the bottom interferometer arm from ‘ π /2’ to ‘0’ results in the construction of a universal NAND rather than an XOR gate: I 1 = I 2 =‘1’ results in O =‘1’ due to the constructive interference, the rest is as in the case of the XOR gate. Moreover, the presented single-chip magnon XOR gate comprises two transistors only, while the CMOS XOR logic gate consists of eight field-effect transistors. Finally, the key advantage of the logic gates based on magnon transistors, that makes it different from any other realization of spin-wave logic [18] , [19] , [20] , [21] , is that the output signal from the gate can be directly sent as an input signal to the next logic gate allowing, in such a way, for the design of all-magnon circuits similar to the integrated circuits in CMOS. The main idea of the manuscript is to show that all-magnon data processing is possible solely within a magnonic system. To demonstrate this experimentally, the proof of concept magnon transistor was developed. Nevertheless, in the final part of the manuscript, we would like to discuss the potential of the magnon transistor from the point of view of practical application. The most crucial questions such as device sizes, operational frequencies and energy consumption are discussed below. The length of the presented magnon transistor demonstrator is 8 mm (distance between the gate and the drain antennas) and a 6-mm long YIG-based magnonic crystal constitutes its largest part (20 periods with 300 μm periodicity). Obviously, a drastic miniaturization of the transistor is required. The first step forward was recently taken by our group [27] when YIG structure sizes were decreased to the micrometre scale (that is, three orders of magnitude comparing with classical YIG structures [10] ). We used e-beam lithography and Ar + etching in order to produce spin-wave conduits of 5 μm width from a 100-nm thick YIG film. The spin-wave propagation length in these conduits is equal to a few tens of microns that is, about ten times better than in analogous metallic ferromagnetic structures. Moreover, it has been shown that the propagation length can be increased up to 1 mm [27] . In order to estimate the minimum length of the magnon transistor, which can be produced on the basis of this microstructured YIG concept, one has to take into account the smallest spin-wave wavelength λ =10 μm that was excited in our studies [27] . This wavelength defines the lattice constant of the magnonic crystal a = λ /2=5 μm for the first band gap. Taking into account the minimum number of periods 10, which ensures an effective magnon localization [38] , the magnon transistor gate of 50-μm length can be produced limiting the transistor’s length. Furthermore, as it was recently shown in ref. 46 , the same technique allows for a further decrease in the width of the magnonic conduit down to hundred nanometre. This, in combination with the decrease in the width of the exciting antenna to 50 nm (in order to operate with spin waves of wavelength λ =100 nm), allows for the miniaturization of the transistor to a size of 500 nm. One more step in the miniaturization can be realized nowadays using, for example, a Helium ion microscope-based technology instead of e-beam lithography. This technique should allow for the fabrication of 5-nm wide antennas. As a result, the transistor will have the length of 50 nm and will operate with magnons of λ =10 nm wavelengths. Finally, the minimum possible size of the transistor is limited by the fundamental minimum spin-wave wavelength λ min in YIG, which is subsequently given by the YIG lattice constant of 1.24 nm. The minimum fundamental length of the magnon transistor of the proposed design is approximately 6.2 nm. It is also important to note that miniaturization also allows for the removal of another drawback of the magnonic devices—the propagation loss of magnons. For example, particularly in our case, the magnon velocity of around 28 km s −1 and the magnon lifetime of 190 ns determine a magnon propagation length to be 5.3 mm. Thus, the amplitude of the spin wave decreases to the value of 0.22 of the initial amplitude after propagation of a source-to-drain distance of 8 mm. However, the situation is completely different for exchange magnons in the nano-scaled magnon transistor described above. In this case, the amplitude will decrease only to a value of 0.997 of the initial amplitude during the 500 nm source-to-drain distance (the calculation is done for magnons of λ =100 nm having the velocity of 1 km s −1 ). Moreover, the efficiency of the four-magnon scattering process of the short-wavelength exchange magnons [43] might be even higher due to the large density of states (see Fig. 3b ). The high operational frequency of the device is another crucial requirement of modern application. In the case of magnon-based devices, the operating frequency is strongly coupled to the frequency of the magnons themselves. In the current experiments, we operate with dipolar magnons of frequencies around 7 GHz. This frequency, however, lies far away from the edge of the Brillouin zone, which determines the maximum magnon frequency. The magnon spectra in YIG measured using neutron scattering show the edge of the first Brillouin zone at about 7 THz [28] , [29] . There are two ways in which the THz band can be reached experimentally. The first one relies on an increase in the applied magnetic field. This way does not seem to be promising since it requires very large magnetic fields (for example, in order to raise the ferromagnetic resonance frequency in YIG up to 1 THz, an external magnetic field around 36 T has to be applied). Therefore, a much more promising method is based on a decrease of the magnon wavelength and goes along with the idea of miniaturization of magnonic elements. Taking into account quadratic dispersion of the short-wavelength exchange magnons, a decrease in the magnon wavelength will result in a drastic increase of their frequencies even in the absence of an external field. Thus, the frequency of magnons of 10-nm wavelength (which can be reached in the course of miniaturization of YIG-based structures) is approximately 0.63 THz even for a very small external field of 5 mT (this field is required for ensuring a single-domain state of YIG films). Furthermore, a high magnon frequency is a necessary but not a sufficient condition for the high operational speed of the magnon devices. In the proposed realization of the magnon transistor, the speed of the four-magnon scattering limits the operational frequency at a level of about 10 MHz. However, an increase of the magnon frequency naturally leads to an intensification of the four-magnon scattering processes: according to the theoretical estimations (see, for example, equation (11.27) in ref. 8 ), the four-magnon relaxation frequency for the exchange magnons scales nearly quadratic with the magnon’s frequency. Thus, we might expect that the increase of the magnon frequency from 7 GHz to 0.7 THz will result in an increase in the operational frequency of the transistor from 10 MHz to 100 GHz. Small energy consumption of a device is another crucial requirement for a modern application. No attempts to decrease the energy consumption of the proposed proof of concept transistor have been made in our studies. However, we can estimate the amount of energy that is consumed in the switching process of the logic output from ‘1’ to logic ‘0’ in our experiments. The easiest way to calculate this energy is to multiply the G-magnon power 25 mW (smallest magnon density required for the switching of the output to ‘0’) with the time 100 ns required for the development of the four-magnon scattering at this power. As a result, we used 2.5 × 10 −9 J to switch a single bit of information while nowadays the standard value for CMOS is around 10 −16 J. However, there are different ways that allows for the decrease in the energy consumption. The most straightforward one is again the miniaturization since the density of the magnons injected into the transistor’s gate, which is required for efficient four-magnon scatterings process, has to be constant. Thus, the decrease in the current sizes of the transistor (5.5 μm × 1.5 mm × 6 mm: the film thickness multiplied with the waveguide width and the magnonic crystal length) to the sizes already reported in ref. 27 (100 nm × 5 μm × 50 μm) will result in a drastic decrease of the energy consumption by six orders of magnitude to 1.2 × 10 −13 J. The next step of the miniaturization to 20 nm × 100 nm × 0.5 μm sizes will lead to a decrease the energy consumption to 4.8 × 10 −18 J, which is two orders of magnitude better than current CMOS values. The last issue, which we would like to discuss here, is the combination of two or more magnon transistors into a magnon circuit. The chip proposed in Fig. 4c seems to be a straightforward and reliable solution for this purpose. The advantages of this chip are that it consists of only one material (YIG in our case), is planar, and the number of the elements that might be produced within the same etching process is practically unlimited. However, one has to keep in mind that in our case the frequencies of S-magnons and G-magnons are different f S ≠ f G . Thus, two kinds of transistors with different magnonic crystal constants a 1 and a 2 might be utilized. The constants a 1 and a 2 can easily be tuned in such a way that f G2 = f S1 and f G1 = f S2 . This approach allows for the combination of an infinite number of magnon transistors in a proper sequence. Finally, it is necessary to note that the data processing based on the usage of Mach–Zehnder interferometers [18] , [19] , [20] results in an decrease in the magnitude of the output signal after the logic gate when compared with the input signal due to a splitting of magnon currents in interferometers. Thus, the combination of a large number of the units requires an intermediate amplification of the signal. At this time, the most promising approaches to realize the amplification are parametric pumping (when the magnonic chip is placed in an external radio frequency field of twice the frequency) [47] applied via contact-less antennas [48] or the spin Hall effect in combination with the spin transfer-torque effect (when the magnonic chip is covered with a metal layer conducting a direct current current) [23] . In conclusion, we have realized a magnon transistor in which the source-to-drain magnon current is controlled by the injection of magnons into the transistor’s gate. The operational principle of the transistor is based on a nonlinear four-magnon scattering process strongly enhanced by the magnonic crystal ensuring high magnon densities at the gate. We have shown that the transistor can be used directly for the designing of logic gates in all-magnon circuits and enables the amplification of signals coded into the magnon density. Although the operational characteristics of the presented insulator-based transistor in its proof-of-principle-type form do not overcome those of CMOS devices, we have demonstrated the realization of the magnon-by-magnon control principle, which is required for data processing on a single magnetic chip. Our analysis shows clear perspectives as it relates to the drastic miniaturization, an increase in the operating frequency, and a decrease in the energy consumption of the device. Thus, the presented transistor is a key element for future particle-less technology, in which information will be carried and processed by magnons rather than by electrons. Magnonic crystal YIG (Y 3 Fe 5 O 12 , YIG) was chosen as a magnetic material for the preparation of a key component of the magnon transistor—the magnonic crystal. YIG is a ferrite (magnetic insulator) with a band gap of 2.85 eV [25] and exhibits the smallest known value for magnetic relaxation of any practical material [10] , [28] . The crystal was designed in the form of a YIG strip with an array of 20 parallel grooves of 0.5 μm depth, 30 μm widths and 270 μm spacings (crystal’s lattice constant a =300 μm) transversely oriented with respect to the spin-wave propagation direction. The grooves were chemically etched with hot ortho-phosphoric acid [33] , [38] on the surface of 5.5-μm thick YIG film grown by liquid-phase epitaxy on a gallium gadolinium substrate in the (111) crystallographic plane. The photolithographic patterning of the magnonic crystal structure was based on a standard photoresist AZ 5214E hardened by ultra-violet baking, which makes it stable against hot 160 °C ortho-phosphoric acid. Spin-wave dispersion characteristics The dispersions have been calculated [49] for a YIG film of 5.5-μm thickness having a saturation magnetization of 139 kA m −1 , an anisotropy field of 3 mT, an exchange constant 3.9·10 −12 J m −1 and an applied bias field of 177 mT. Please note that the real number of spin-wave modes in the film is much higher since the magnons are allowed to propagate at different angles and, correspondingly, have different dispersion relations, which are not shown here for simplicity [8] , [50] . The lowest (zeroth) magnon mode with a uniform distribution of the magnetization precession over the film thickness, shown in black bold in Fig. 3a , has a maximal efficiency for excitation and detection by the microstrip antenna [10] . Therefore, the originally injected S-magnons (blue-filled circle) as well as G-magnons (red-filled circles) are located on the lowest magnon mode. How to cite this article: Chumak, A. V. et al. Magnon transistor for all-magnon data processing. Nat. Commun. 5:4700 doi: 10.1038/ncomms5700 (2014).